Spider genomes provide insight into composition and evolution of venom and silk Spiders are ecologically important predators with complex venom and extraordinarily tough silk that enables capture of large prey. Here we present the assembled genome of the social velvet spider and a draft assembly of the tarantula genome that represent two major taxonomic groups of spiders. The spider genomes are large with short exons and long introns, reminiscent of mammalian genomes. Phylogenetic analyses place spiders and ticks as sister groups supporting polyphyly of the Acari. Complex sets of venom and silk genes/proteins are identified. We find that venom genes evolved by sequential duplication, and that the toxic effect of venom is most likely activated by proteases present in the venom. The set of silk genes reveals a highly dynamic gene evolution, new types of silk genes and proteins, and a novel use of aciniform silk. These insights create new opportunities for pharmacological applications of venom and biomaterial applications of silk. Spiders (Araneae) are an order of Arachnida (Chelicerata) with >44,500 described extant species [1] . They occupy habitats from the most arid deserts to the extreme Arctic, owing to broad physiological adaptations and a diverse behavioural repertoire. One main clade is the mygalomorphs containing tarantula-like spiders that are ground dwelling sit-and-wait predators that subdue passing prey; another clade is the araneomorphs that have diversified greatly to occupy all types of above-ground habitats, and evolved sophisticated capture webs to intercept flying insects [2] . The significant ecological impact of spiders as predators, for example, in top-down control of insects and pests in natural and managed ecosystems [3] , [4] , [5] , is tightly linked to the use of lethal venom to subdue prey, which in combination with the production of silk webs facilitates efficient prey capture at minimum energetic cost. These adaptations allow spiders to catch prey as much as seven times their own body weight [6] , an astonishing ratio for predators across all taxa. Spider venom attracts wide interest because of its biochemical and structural properties [7] , [8] , pharmacological applications [9] and the pathophysiological impact on humans following bites from species such as the redback, black widow and brown recluse spiders. Venom neurotoxins target specific types of insect ion channels and receptors and have wide applied potential as insecticides in pest control [10] . Spider silk is characterized by incredible strength and elasticity, which has prompted intensive research into its biochemical and physical properties [11] , [12] , and industrial interest in its biomaterial application [13] . Complete sequences of spider genes are required to facilitate the identification of venom proteins and peptides, and to progress the active research field of silk bioengineering. The most successful taxa of chelicerates are spiders and mites/ticks (Acari) in terms of both species numbers and ecological and economic importance. However, of the chelicerates only Acari genomes are available. To advance our understanding of genome evolution in arthropods, it is important to include other chelicerates to fill the vast phylogenetic gap from Acari to insects and crustaceans. Genomic information from spiders has the potential to resolve phylogenetic relationships within the arthropods such as the long-standing controversy on whether Acari are monophyletic or paraphyletic [14] . Genomic information is also needed to progress our understanding of the evolution of development [15] , [16] and the body plan of metazoans [17] , [18] . We report the assembled genome of the araneomorph African social velvet spider, Stegodyphus mimosarum , and a draft assembly of the mygalomorph Brazilian white-knee tarantula, Acanthoscurria geniculata . We use transcriptomics and large-scale proteomic experiments for gene annotation, and perform in-depth analyses of venom and silk proteomes. The two species represent major araneid clades and are important in evolutionary and proteomic research. The velvet spider is one of very few cooperative species, and it is becoming a model for studying sociality and inbreeding mating systems [19] . The tarantula is a model for studying venom proteins, and is particularly well suited for studies of extra-oral digestion and proteolytic enzymes. Genome assembly and gene annotation A de novo assembly of the velvet spider was generated from 91 × coverage sequencing of paired end and mate pair libraries (up to 20 kb insert sizes) from the highly inbred social velvet spider S. mimosarum ( Supplementary Note 1 ). 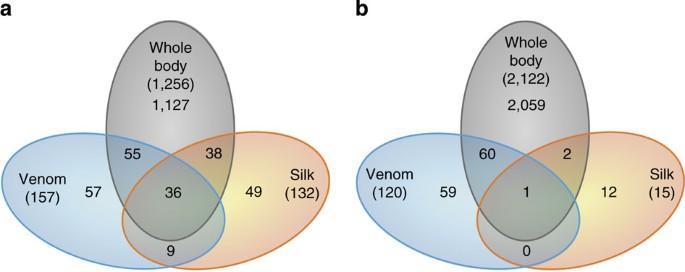Figure 1: Proteomics. Venn diagrams with number of identified proteins based on 194 LC-MS/MS analyses (Supplementary Table 3). The silk analyses are based on in-solution trypsin digestion, while the body analyses are based on in-gel trypsin digestion. The venom analyses are based on a combination of the two methods. (a) Velvet spider. (b) Tarantula. The low heterozygosity of 0.02% allowed efficient assembly into contigs and scaffolds spanning 2.55 Gb ( Table 1 ). High-quality single-nucleotide polymorphisms (SNPs) 1.09 million were identified from mapping back to scaffolds ( Table 1 ). Table 1 Genome statistics for the velvet spider and tarantula. Full size table The gene content of the velvet spider genome was analysed by constructing gene models supported by three lines of evidence using our in-house developed pipeline for the process ( Supplementary Figs 1 and 2 ; Supplementary Table 1 ). The evidence include transcriptomics and proteomics, as well as homology to known proteins. Identification of gene products at the protein level is strong evidence for a predicted gene and demonstrates that the gene is functional. Although this procedure is rarely used in studies reporting on de novo assemblies of genomes, it provides a gene set of very high quality. Our final gene set includes 27,235 protein-coding gene models, of which 70% could be functionally annotated from comparative analysis. 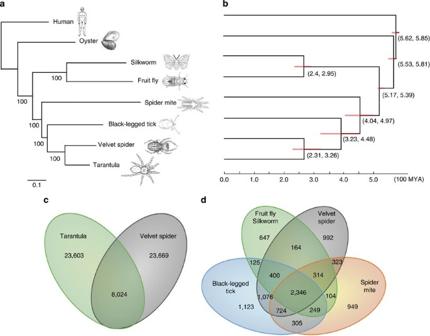Figure 2: Comparative genomics. (a) Phylogenetic tree based on the amino-acid sequence of 452 one-to-one orthologous genes in eight species. (b) Estimated divergence times using a relaxed molecular clock and fossil calibration time ranges. Red bars are 95% credibility intervals. (c) The 1-1 orthologous genes between the two spider species. (d) The number of gene families shared among the species using the TreeFam classification scheme among spiders, mites, ticks and insects. Approximately 400 gene models with no homology to known proteins were supported by proteomic evidence and these are strong candidates for ‘spider’-specific proteins ( Table 1 ; Supplementary Table 2 ). The exon-intron structure, unlike other arthropod genomes, is characterized by short exons and long introns very similar to the human genome ( Table 1 ). This suggests that similar selective forces on genome size are operating in spiders and mammals. After generating this gene set, we used mass spectrometry (MS) data related to the velvet spider to query the final gene set identifying 157 proteins from venom, 132 proteins from silk and 1,256 proteins from body tissue. In total, 1,371 proteins were identified in the velvet spider ( Fig. 1a ; Supplementary Data 1 ). Figure 1: Proteomics. 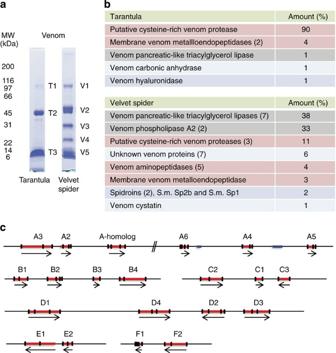Figure 3: Venomics. (a) Coomassie-blue-stained SDS-gel of venom from tarantula and velvet spider, respectively, (Supplementary Fig. 16). The major protein(s) in the bands are: T1, membrane venom metalloendopeptidase-a; T2, putative cysteine-rich venom protease; T3, genicutoxin A1; V1, membrane venom metalloendopeptidase and venom aminopeptidase-a; V2, venom pancreatic-like triacylglycerol lipase-a and c; V3, cysteine-rich venom protease-a; V4, venom phospholipase A2-a; and V5, S.m. Sp2b. In addition to S.m. Sp2b, the V5 band also contains several protoxins. The composition of the visual blue bands was specifically interrogated using the relevant LC-MS/MS analyses of bands from the gels shown inSupplementary Figs 4 and 5. The data are a sub-fraction of the data shown inSupplementary Data 1 and 2, where the merged result of LC-MS/MS analyses of gel bands from a complete gel lane is presented. (b) The table summarizes quantitative analyses of venom proteins, excluding protoxins (mainly present in the lower bands on the gel inFig. 3a). The reason to exclude the protoxins from this analysis is described in theSupplementary Note 2. The proteases are shown in red, the lipases in grey and the other proteins in shades of blue. Numbers in parentheses refer to the number of variants of the particular protein that were quantified. Individual proteins constituting <1% of the venom protein content are not included. These quantitative LC-MS/MS analyses are based on a gel-free approach and extracted ion chromatography (XIC). The table is an extract of the full quantitative analyses (Supplementary Data 7 and 8). (c) The genomic localization of the protoxin families in the velvet spider, the stegotoxins, is depicted. The letters (A–F) indicate the family, based on sequence similarities, and the numbers distinguish between the different toxins in the same family (Supplementary Note 2). The ‘A-homologue’ refers to a sequence homologous with the A-family of toxins, but without proteomic support. The arrows indicate the direction of transcription. Introns are shown in red and coding sequences in black. In the A-family cluster, two non-related predicted protein-coding genes are present. These are shown as blue rectangles. The figure shows that toxins with sequence similarities cluster on the genome. Venn diagrams with number of identified proteins based on 194 LC-MS/MS analyses ( Supplementary Table 3 ). The silk analyses are based on in-solution trypsin digestion, while the body analyses are based on in-gel trypsin digestion. The venom analyses are based on a combination of the two methods. ( a ) Velvet spider. ( b ) Tarantula. Full size image The size estimate of the tarantula genome based on k-mer analysis is >6 Gb and we sequenced at 40 × coverage from a single female A. geniculata using a similar combination of paired end and mate pair libraries as for the velvet spider. The combination of lower coverage, larger genome and 30 times higher heterozygosity (0.34%) resulted in a very fragmented assembly ( Table 1 ). Therefore, the gene set was based on de novo transcript assembly and proteomics. We collapsed transcript assemblies from the body (abdomen and head), an opisthosomal gland and venom gland to generate the final tarantula sequence set of ~70,000 transcripts. To build a comprehensive mygalomorph spider proteome, we sequenced proteins from venom, thorax, abdomen, haemolymph and silk by liquid chromatography-tandem mass spectrometry (LC-MS/MS) ( Supplementary Methods ; Supplementary Table 3 ). These data were used to query the final tarantula transcript database identifying 120 proteins in venom, 15 proteins in silk and 2,122 proteins from body fluid and tissue samples. In total, we identified 2,193 tarantula proteins, which to our knowledge is the largest spider proteome ( Fig. 1b ; Supplementary Data 2 ). The exon-intron structure was estimated by mapping gene models back to the fraction of scaffolds >100 kb and due to the fragmented assembly, this is likely to be an underestimate of the average intron length in tarantula, but still, introns were found to be longer than those of the velvet spider ( Table 1 ). Nucleotide and amino-acid sequences of proteins of interest from any of the two spiders can be found in the supplementary fasta-files ( Supplementary Data 3–6 ), which include all released sequences. The files are sorted according to accession numbers, and these accessions numbers are also used in Supplementary Data 1,2,7–9 . Comparative genomics The repeat content estimate from repeat scout analysis identifying easily recognizable repeats of the velvet spider genome is similar to that of the human genome ( Table 1 ; Supplementary Tables 4 and 5 ). Repeats are more difficult to detect in the fragmented tarantula assembly. To evaluate the effect of lower coverage on repeat content, we downsampled the velvet spider sequences to obtain a similar quality assembly as in tarantula and found that the repeat content estimate decreased by 9%. By extrapolating from the repeats identified in the tarantula genome (57%), we therefore estimate a repeat content of ~60% in tarantula. This result suggests that repeat expansion is at least part of the reason for a large genome size. Blasting the longest tarantula contigs against themselves does not identify recent genome duplication. However, owing to the large divergence time (see below) of the two species there may not be a single, easily identifiable reason for genome size differences. There is no evidence for a isochore structure but a general difference in GC content is observed (~35% in velvet spider and ~40% GC in tarantula). From a comparison of the velvet spider gene set and the tarantula transcripts, 452 genes had one-to-one orthologous genes in the two spider species, and in selected species of arthropods, oyster and human. A phylogenetic tree was reconstructed from the amino-acid sequences of these genes using PhyML [20] ( Fig. 2a ). We found strong bootstrap support for spiders and ticks as sister groups with mites as the outgroup. This result strongly supports recent claims that mites and ticks do not form a monophyletic group (Acari) [21] as has previously been thought [22] . Phylogenetic dating using a relaxed molecular clock dates separation of velvet spider and tarantula at 270 MY, ticks and spiders at 390 MY, and mites and spiders at 455 MY ( Fig. 2b ), confirming the deep split of velvet spider and tarantula within the chelicerates. Reciprocal BLAST analysis identified 8,024 one-to-one orthologous genes between velvet spider and tarantula ( Fig. 2c ), which have a broad distribution of amino-acid divergence ( Supplementary Fig. 3 ). We also used gain or loss of gene families (based on the Treefam classification) as phylogenetic characters. We show that ticks share many more gene families with the velvet spider (1,476) than mites share with the velvet spiders (637) ( Fig. 2d ). If we assume that the probability of loss or gain of each gene family is proportional to separation time, this analysis lends additional support to the results of the phylogenetic relationships ( Fig. 2a ). Figure 2: Comparative genomics. ( a ) Phylogenetic tree based on the amino-acid sequence of 452 one-to-one orthologous genes in eight species. ( b ) Estimated divergence times using a relaxed molecular clock and fossil calibration time ranges. Red bars are 95% credibility intervals. ( c ) The 1-1 orthologous genes between the two spider species. ( d ) The number of gene families shared among the species using the TreeFam classification scheme among spiders, mites, ticks and insects. Full size image To identify the genomic properties that make a spider unique, we identified Treefam gene families that are expanded in both spider species [23] , [24] . Owing to the fragmented tarantula assembly, we focus only on gene families that show very conspicuous expansions in both spider species ( Supplementary Data 10 ). Among these families are astacin-like metalloproteases, which previously have been linked to extra-oral digestion [25] , a key feature of spiders, and of venom [26] . Half of the astacin-like metalloproteases sequences that we present are supported by proteomic evidence ( Supplementary Data 1 and 2 ). We mainly identify the enzymes in the analyses of ‘whole-body’ samples (19 astacin-like metalloproteases are identified in velvet spider and 10 in the tarantula), which is consistent with the proteases being expressed in the digestive organs. Except for two proteases, identified in velvet spider venom at low concentrations, the astacin-like metalloproteases are not present in venom from the two spiders. Thus, our data indicate that this expanded family of proteases primarily plays a role in the extra-oral digestion, but future proteomics studies targeting digestive fluid from spiders are needed to confirm the presence of these proteases in digestive fluid. Venomics Comparing the venom protein profiles of the two spider species by gel electrophoresis reveal that they both contain a large fraction of relatively small proteins below 10 kDa, likely to include the cysteine-rich peptide toxins ( Fig. 3a ; Supplementary Figs 4 and 5 ). These are known to mediate the neurotoxic effects of venom [27] . These toxins are small proteins containing a signal peptide, a propeptide and the sequence encoding the mature toxin [28] . However, the conversion from the proform to the active toxin has not previously been described and putative proteases involved in the process have never been identified. Our analysis indicates that the most abundant spider venom proteases are involved in the activation of venom protoxins (details below). Figure 3: Venomics. ( a ) Coomassie-blue-stained SDS-gel of venom from tarantula and velvet spider, respectively, ( Supplementary Fig. 16 ). The major protein(s) in the bands are: T1, membrane venom metalloendopeptidase-a; T2, putative cysteine-rich venom protease; T3, genicutoxin A1; V1, membrane venom metalloendopeptidase and venom aminopeptidase-a; V2, venom pancreatic-like triacylglycerol lipase-a and c; V3, cysteine-rich venom protease-a; V4, venom phospholipase A2-a; and V5, S.m. Sp2b. In addition to S.m. Sp2b, the V5 band also contains several protoxins. The composition of the visual blue bands was specifically interrogated using the relevant LC-MS/MS analyses of bands from the gels shown in Supplementary Figs 4 and 5 . The data are a sub-fraction of the data shown in Supplementary Data 1 and 2 , where the merged result of LC-MS/MS analyses of gel bands from a complete gel lane is presented. ( b ) The table summarizes quantitative analyses of venom proteins, excluding protoxins (mainly present in the lower bands on the gel in Fig. 3a ). The reason to exclude the protoxins from this analysis is described in the Supplementary Note 2 . The proteases are shown in red, the lipases in grey and the other proteins in shades of blue. Numbers in parentheses refer to the number of variants of the particular protein that were quantified. Individual proteins constituting <1% of the venom protein content are not included. These quantitative LC-MS/MS analyses are based on a gel-free approach and extracted ion chromatography (XIC). The table is an extract of the full quantitative analyses ( Supplementary Data 7 and 8 ). ( c ) The genomic localization of the protoxin families in the velvet spider, the stegotoxins, is depicted. The letters (A–F) indicate the family, based on sequence similarities, and the numbers distinguish between the different toxins in the same family ( Supplementary Note 2 ). The ‘A-homologue’ refers to a sequence homologous with the A-family of toxins, but without proteomic support. The arrows indicate the direction of transcription. Introns are shown in red and coding sequences in black. In the A-family cluster, two non-related predicted protein-coding genes are present. These are shown as blue rectangles. The figure shows that toxins with sequence similarities cluster on the genome. Full size image The overall venom protein compositions of the two spiders are distinct with a single dominating band around 45 kDa in tarantula and a more complex pattern in the velvet spider ( Fig. 3a ; Supplementary Figs 4 and 5 ). A relative quantification of venom proteins was performed using MS-based label-free quantification based on extracted-ion chromatography (XIC) ( Fig. 3b ; Supplementary Data 7 and 8 ). For these analyses venom proteins were denatured, reduced, alkylated and digested with trypsin in-solution. Only proteins were included in this analysis, as the small protoxins are less suitable for the chosen quantitative approach, as described in the Supplementary Note 2 . The quantification showed that the dominating band (T2) on the gel constituted >90% of the total protein (exclusive protoxins) and is homologous to the cysteine-rich secretory protein 3 (CRISP3). CRISP3 is also referred to as venom allergen and is found in venom of, for example, cone snail, wasp, snake and lizard [29] , [30] . In the cone snail, the protein functions as a serine protease and cleaves the propeptide of the snails’ cysteine-rich peptide-toxins (‘conotoxins’) [29] . The finding of the orthologous tarantula CRIPS3-like protein in the tarantula venom, and the sequence similarities between toxins from the two species, suggest that the protein similarly functions as a protoxin-converting enzyme and we name it ‘putative cysteine-rich venom protease’. Previous studies identified the major protein component of tarantula venom as a hyaluronan-degrading enzyme (hyaluronidase) [31] , [32] , [33] . We also identify a hyaluronidase, however, from quantitative MS analysis, in much lower abundance than the putative cysteine-rich venom protease ( Fig. 3b ; Supplementary Data 7 ). In previous studies, the CRISP3-like protein was probably overlooked because of the hyaluronidase activity-based assays used combined with similarity in size of the two proteins [31] , [32] , [33] . A CRISP3 homologue was also found in the venom of the velvet spider ( Fig. 3a,b ; Supplementary Data 8 ). In contrast to tarantula, three different isoforms of this protein were identified, and comparison with the cone snail CRISP suggests that they are all proteases. Of the 13 quantified proteins in tarantula venom, four additional putative proteases were identified, but at a much lower concentration than the putative cysteine-rich venom protease ( Supplementary Data 7 ). One of the proteases is named ‘venom proprotein convertase’ and is homologous to other proprotein convertases know to process precursor proteins such as prorenin, progastrin and proinsulin into their biological active products. In general, proprotein convertases cleave after arginine, which is also the required activity for activation of the main part of spider protoxins, and the venom proprotein convertase is also likely to be involved in processing of protoxins. Furthermore, two ‘membrane venom metalloendopeptidases’ were identified. They belong to the peptidase family M13 that is characterized by acting on substrates smaller than proteins, which is also consistent with a role in toxin activation. The M13 family includes the specific endothelin-converting enzymes that process the preform of the peptide hormone endothelin and generates the active product. In the velvet spider venom, 11 of 33 quantified proteins were proteases based on sequence homology ( Supplementary Data 8 ). Among the 11 proteases are three isoforms of the putative cysteine-rich venom proteases that are likely to be involved in activation of toxins, as described above. The four most abundant proteases in velvet spider venom are the three isoforms and a putative protease with homology to the peptidase family M13. Thus, many of the proteases in velvet spider venom could be involved in toxin activation. Venom proteases have previously been suggested to cause tissue destruction and thus facilitate toxin penetration or to be involved in the initial extra-oral digestion of the prey [34] . While this function could not be excluded, the findings in this study indicate that these venom proteases primarily play a role in the activation of protoxins. Our analysis also shows that the proteases in venom are different from the proteases previously identified in the digestive fluid of an araneomorph spider, namely the previously mentioned astacin-like metallopeptidases [25] . The protease fraction constitutes a smaller proportion of venom proteins in the velvet spider compared with tarantula ( Fig. 3b ), and the two species also differ in the number of lipases, as nine (of 33) were identified in the velvet spider and only one (of 13) in tarantula ( Fig. 3b ; Supplementary Data 7 and 8 ). These lipases were very abundant in the velvet spider, where two lipases constituted >70% of the venom proteins, while only accounting for ~1% of the venom proteins in tarantula. Phospholipase A2 enzymes have previously been reported in the venom from sea anemones, bees, lizards, scorpions, snakes and other spider species [35] , and were shown to function as neurotoxins, myotoxins and anticoagulants in snakes [36] . In contrast, the pancreatic-like lipases found in both spiders have, to our knowledge, not previously been identified in venom. The large difference in lipase concentration between the two spiders suggests different toxic strategies. The majority of the remaining larger proteins found in the venom from the two species are homologues of known enzymes, except for the interesting identification of two spidroin proteins (S.m. Sp2b and S.m. Sp1), usually involved in structural properties of spider silk ( Fig. 3b ). This is not the result of contamination, since the spidroins were highly abundant in the venom and were identified in all biological and technical replicates ( Supplementary Data 1 and 8 ). It is not known whether they form fibres in the venom, but the S.m. Sp2b protein (complete protein ~500 kDa) is fragmented and only identified in the lower part of the SDS-polyacrylamide gel electrophoresis (PAGE) gel (~25 kDa). The biological function of spidroins in velvet spider venom and the prevalence of this phenomenon among other spider species remain to be investigated. Spider venom generally contains high concentrations of smaller cysteine-rich proteins dominated by knottins, which cause their neurotoxic effects [37] . These proteins have insecticidal [10] and pharmaceutical potential and currently five therapeutic leads exist [38] . Using a targeted approach ( Supplementary Note 2 ), 78 knottin-encoding transcripts were identified in the tarantula transcriptome. A semi-quantitative MS analysis ( Supplementary Note 2 ) indicates that the most abundant of the cysteine-rich protoxins in tarantula is similar to the Hainantoxin-XVIII family from the Chinese tarantula ( Haplopelma hainanum ) [28] ( Supplementary Data 7 ). In the velvet spider genome, we identified 51 knottin-like protoxin-encoding genes, 28 of these were supported at the transcriptomic level, 26 at the protein level and 20 by both methods ( Supplementary Note 2 ; Supplementary Data 9 ). All toxins with protein evidence were aligned and clustered in nine families based on sequence similarities ( Supplementary Fig. 6 ). These families were named Stegotoxin family A-I with Stegotoxin A7 as the most abundant ( Supplementary Data 8 ). All families, except Stegotoxin-C , contain a propeptide sequence. The protease(s) that activates the protoxins seems to be specific for arginine in the P1 position, since all toxins have an arginine residue at the C-terminal end of the propeptide ( Supplementary Fig. 6 ). Subsequently, we explored the gene structure and genome localization of these toxins, demonstrating that the protoxins contained between two and five introns ( Supplementary Data 9 ). The exon-intron structure showed that the mature peptide was based on only one exon ( Supplementary Fig. 6 ), and the genome localization shows that similar sequences cluster on the same scaffold. This indicates that these toxin families evolved by segmental duplication in adjacent regions such as those found in the scorpion Mesobuthus martensii [39] , enabling further diversification by molecular evolution and gene shuffling ( Fig. 3c ). Silkomics We combined the assembled genomes and transcriptomes with proteomic data of spider silk to identify the genetic basis and quantify the expression of the complete set of silk genes. Spider silk fibres are produced by glands in the ventral part of the opisthosoma, and structural proteins of silk are encoded by members of a single gene family, the spidroin genes [40] . Mygalomorph spiders are considered to have a single or a few undifferentiated glands, however, during the evolution of the araneomorph spiders, their glands have differentiated into specialized organs producing specialized silk types [41] , [42] . Shared among araneomorphs are major and minor ampullate-, piriform- and aciniform glands, whereas the tubiliform gland evolved in the common ancestor of entelegyne spiders [43] , a subgroup of araneomorphs. A typical spidroin consists of non-repetitive terminal-folded domains (N- and C-terminal domain) and a central repetitive core region [44] , [45] . Repeats are typically highly conserved within each spidroin, but differ among spidroin types [46] . The physical properties of silk fibres depend on the amino-acid sequence, but also on the spinning conditions, including temperature, humidity and spinning speed [47] . In the velvet spider, a high number of spidroins were identified showing considerable diversity ( Fig. 4a ). We performed phylogenetic analyses of both the N- and C-terminal domains of the putative spidroin sequences in the velvet spider and of all previously sequenced spidroin sequences for classification. Most of the spidroin types form phylogenetic groups across all species providing high support for the classification ( Supplementary Fig. 7 ). However, the major and minor ampullate spidroins show a more scattered signal. We therefore investigated the amino-acid content and repeat motifs in detail. The complete putative major ampullate spidroin sequences showed consistently higher glycine and alanine content compared with the putative minor ampullate sequence ( Supplementary Fig. 8 ). Furthermore, all the putative major ampullate spidroins contain the characteristic poly-A runs, GGX and GA motifs of previously published major ampullate spidroins ( Supplementary Fig. 9 ). In addition, the putative minor ampullate sequence differs from the putative major ampullate sequences by containing non-repetitive regions flanking the repetitive core region, which was also found in previously studied species [48] . 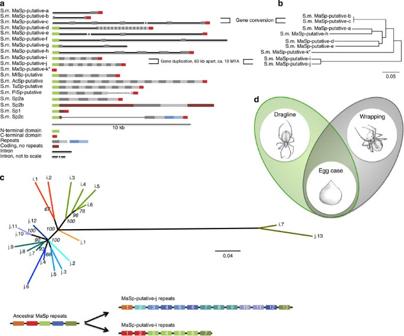Figure 4: Silk genes in the velvet spider. (a) Schematic overview of exon-intron and repeat structure of the identified silk genes. The repeats from a single locus share evolutionary history and are easy to align, except for S.m. Sp2c that consists of two sets of repeats (grey and blue) with different evolutionary histories. S.m. PiSp consists of sequences obtained from two scaffolds. PCR verified that they come from the same locus. (b) The evolutionary history of the major ampullate C-terminal domain, including the recent events of gene conversion, whole-gene duplication (~10 MYA) and pseudogenization* (Supplementary Note 3). Scale bar represents number of nucleotide differences per site. (c) Major ampullate repeat evolution over ~10 MY since a whole-gene duplication. The evolutionary relationship of repeats from two recently duplicated loci is depicted by a phylogenetic tree and repeat structures. Similar coloured repeats are evolutionarily most related. Scale bar represents the number of nucleotide differences per site. (d) Use of aciniform silk in the velvet spider compared with previously studied species that use aciniform silk to wrap their prey. Velvet spiders do not wrap their prey, but use aciniform silk for dragline silk in combination with major ampullate silk. Velvet spiders also use aciniform silk for egg case construction as do previously studied species. Figure 4: Silk genes in the velvet spider. ( a ) Schematic overview of exon-intron and repeat structure of the identified silk genes. The repeats from a single locus share evolutionary history and are easy to align, except for S.m. Sp2c that consists of two sets of repeats (grey and blue) with different evolutionary histories. S.m. PiSp consists of sequences obtained from two scaffolds. PCR verified that they come from the same locus. ( b ) The evolutionary history of the major ampullate C-terminal domain, including the recent events of gene conversion, whole-gene duplication (~10 MYA) and pseudogenization* ( Supplementary Note 3 ). Scale bar represents number of nucleotide differences per site. ( c ) Major ampullate repeat evolution over ~10 MY since a whole-gene duplication. The evolutionary relationship of repeats from two recently duplicated loci is depicted by a phylogenetic tree and repeat structures. Similar coloured repeats are evolutionarily most related. Scale bar represents the number of nucleotide differences per site. ( d ) Use of aciniform silk in the velvet spider compared with previously studied species that use aciniform silk to wrap their prey. Velvet spiders do not wrap their prey, but use aciniform silk for dragline silk in combination with major ampullate silk. Velvet spiders also use aciniform silk for egg case construction as do previously studied species. Full size image Since the classified spidroins are based on indirect evidence, and not on gland-specific expression (see a recent study for evidence of non-gland-specific expression of some spidroin types [49] ), we named them ‘putative’. On the basis of the classification, we identified one copy of each of the aciniform, tubiliform, piriform and minor ampullate spidroin sequences, and remarkably 10 copies of the major ampullate spidroins. In addition, four novel spidroin sequences were discovered ( S.m. Sp1 and S.m. Sp2a-c ), where S.m. Sp1 groups with flagelliform spidroins (though not closely), and the remaining three sequences group together ( Supplementary Fig. 7 ). However, the flagelliform spidroin is not expected to be found in cribellate silk such as that of the velvet spider [50] , and the absence of a repeat structure and the short length (~1,100 bp) of the S.m. Sp1 locus also differs significantly from the flagelliform loci previously described. This deviation from a typical spidroin repeat structure is also found in S.m. Sp2b and S.m. Sp2c . Two repeats were identified in the central part of the S.m. Sp2b locus, but most of the sequence between the terminal domains is not repetitive. S.m. Sp2c has four repeats that lack an obvious common history; instead S.m. Sp2c consists of two sets of repeats with different evolutionary histories ( Fig. 4a ). In contrast, the structure of S.m Sp2a resembles a typical spidroin with N- and C-terminal domains bracketing the usual repeat structure. The transcriptomic and proteomic analyses of ‘whole web’, egg case and dragline silk, respectively, demonstrated functional support for all silk genes except one ( S.m. MaSp-putative-k ) ( Supplementary Table 6 ). The repeat-structure and exon-intron structures of major ampullate spidroin copies are rather heterogeneous. One sequence ( S.m. MaSp-putative-e ) has no obvious repeats, but has an internal exon with repeat-like amino-acid composition, while one sequence shows 28 repeats ( S.m. MaSp-putative-d ) ( Supplementary Table 7 ). At least six of the major ampullate genes contain introns ( Fig. 4a ). The major ampullate sequences form a monophyletic group to previously published spidroin sequences ( Supplementary Fig. 7 ; Supplementary Table 8 ), and document highly dynamic evolution, exemplified by recent gene evolution events of the major ampullate spidroins: one whole-gene duplication ( S.m. MaSp-putative-i and S.m. MaSp-putative-j , about 10 MYA) ( Fig. 4b ), gene conversion of a C-terminal domain ( S.m. MaSp-putative-b and S.m. MaSp-putative-c ) ( Fig. 4b ; Supplementary Fig. 10 ) and by a major ampullate spidroin ( S.m. MaSp-putative-k ) that probably lost its function recently (maximum 7 MYA) ( Fig. 4b ; Supplementary Note 3 ). Owing to recent common ancestry of S .m. MaSp-putative-i and S.m. MaSp-putative-j their repeat sequences are still easily alignable, and analysing their evolution reveals dynamic processes of both loss and duplication of the repeats ( Fig. 4c ). Proteome analyses of dragline and egg case silk reveal multiple functions of aciniform silk in the velvet spider. Tubiliform and aciniform silk are used to build the egg case in the velvet spider, similar to orb-weaving spiders [51] , [52] . In contrast, dragline silk is composed of major ampullate and aciniform spidroins ( Supplementary Data 8 ). This differs from the current understanding that major ampullate spidroins alone make up the dragline silk ( Fig. 4d ; Supplementary Data 8 ). The diversity of the repeat sequences in the aciniform silk is quite high in the velvet spider (~79% identity), in contrast, diversity of aciniform repeats in the widow spider Latrodectus was shown to be very low (~99% identity) [53] . In addition to spidroins, >100 proteins are identified in the analysed silk ( Supplementary Data 1 ). Among the most abundant proteins are several hydroxyacid oxidase-like proteins, peroxinectin and a number of unknown proteins. A large spidroin-like protein with high glycine (45%) and alanine (26%) content was detected in all three silk samples (named ‘silk-related protein’). It has an obvious repetitive structure, but does not seem to belong to the spidroin family, based on lack of similarity of the amino-terminal domain. It has long internal regions of GA-repeats with some of the alanines being replaced by leucine or valine in an irregular pattern. A blast analysis shows that the repetitive region is somewhat similar to the repetitive region of a silkworm silk gene. This does not necessarily imply an evolutionary history of this gene and silkworm silk genes, but may merely be due to convergent evolution of an ensemble motif. In the tarantula transcriptome, we identify 12 sequences with similarity to published spidroins based on blast. Under the assumption of repeat conservation within loci, these partial sequences likely represent up to seven distinct loci ( Supplementary Fig. 11 ; Supplementary Table 9 ). It is only possible to identify a small fraction of these sequences in the genome scaffolds, except for A.g. Spidroin-5 , which is located in a single scaffold. This sequence contains both N- and C-terminal domains, but no obvious repetitive sequence in between, and does not include introns. A.g. Spidroin-1,-2,-4 and -5 all have proteome support from analyses of tarantula silk. A.g. Spidroin-3,-6 and -7 show blast similarity to repetitive regions of previously reported mygalomorph spidroins. They are short sequences with no N- or C-terminal domain sequences. Fewer spidroin loci were found in our study than reported in other mygalomorph species [46] , [54] . The silk gene composition of the tarantula described here is not as complete as for the velvet spider, but our results suggest that the silk gene composition in mygalomorph spiders is far less complex than in araneomorph spiders [55] . This is consistent with the evolution of functionally more diverse silk and silk use by araneomorph spiders, for example, in elaborate prey capture webs and less diverse silk use in tarantula spiders. In line with this, fewer non-spidroin proteins (nine) were associated with tarantula silk ( Supplementary Data 2 ). Research on functional and evolutionary biology of spiders has been limited by an almost complete lack of DNA sequence data. We present the first genome sequence of the araneomorph velvet spider and a fragmented genome sequence of the mygalomorph tarantula. The high heterozygosity, high repeat content and large genome size effectively preclude a high quality assembly of the tarantula by Illumina-sequencing approaches. Genome annotation was aided by large-scale transcriptome and proteome data, providing functional support to predicted gene models, and immediately documenting that genes are protein coding. The exon-intron structure of the spider genome, unlike other arthropod genomes, is characterized by short exons and long introns very similar to the human genome. The inclusion of spider genomes in phylogenetic analysis of chelicerates shows that Acari is polyphyletic by demonstrating that ticks group with spiders and not with mites. In contrast to the previous approaches, where MS mainly was used for de novo sequencing of purified peptide toxins, the high-quality sequence databases provided in the present study facilitate fast and high-throughput LC-MS/MS-based analyses of spider venom. Analyses of spider venom show that both spider species contain a large repertoire of cysteine-rich peptides, which most likely mediates the toxic effects of venom. While it was previously suggested that venom proteases cause tissue destruction to facilitate toxin penetration or are involved in the initial digestion of the prey [34] , we suggest the main function of venom proteases is to process and activate protoxins, because of their homology to proteases involved in the activation of precursor proteins. The two spider species have very different venom protein composition, where lipases are nearly absent in tarantula but represent >70% of the protein fraction in velvet spider venom. In tarantula, a putative protease with homology to CRISP3, a venom allergen found in cone snail, wasp, snake and lizard, constitutes >90% of the venom’s protein fraction. The spider genome facilitates the first complete study of silk genes and their functionality. We find that the composition of velvet spider silk is highly diverse and complex. Two new findings are: (1) the dragline silk of the velvet spider is composed of at least two types of spidroins, major ampullate and aciniform spidroins, and (2) four novel and related spidroin sequences are identified. Our data reveal very dynamic evolution of major ampullate genes, including recent duplication, deletion and gene conversion. Sample collection and genome sequencing A single velvet spider nest was collected in South Africa (GPS position: 29° 39′ 16.46″ S, 30° 27′ 35.55″ E). DNA for short-insert libraries (250, 500, 2,000 and 5,000 bp) was extracted from whole bodies (a single spider for each library). DNA for long insert libraries (10,000 and 20,000 bp) was extracted from a pool of 100 spiders. A single female tarantula was used for DNA extraction. DNA for both short- and long-insert libraries (250, 500, 2,000, 5,000, 10,000 and 20,000 bp) was extracted from soft abdomen tissue. See Supplementary Methods for details on DNA extractions. All libraries were sequenced on Illumina Hiseq 2000. We generated a total of about 361-Gb of data, and 264 Gb (91 × coverage) was retained for assembly after filtering out low quality and duplicated reads for the velvet spider, and about 344 Gb and 255 Gb (40 × coverage) was retained for assembly after filtering out low quality and duplicated reads for the tarantula. For summary, see Supplementary Tables 10 and 11 . Transcriptome sequencing The velvet spider RNA was extracted from a mix of three whole bodies, and a mix of ~100 venom glands. Before library construction, the venom gland complementary DNA pool was normalized. From the tarantula, three pools of total RNA were extracted from different tissues for sequencing: ‘Whole body’, two venom glands and an opisthosomal gland. See Supplementary Methods for details on gland dissections. For the ‘whole-body’ transcriptome tissue from six tarantula individuals, including two fasting spiders, two spiders that were fed with mice and killed after 12 h and two spiders that were fed with mice and killed after 48 h, were used. Tissue was pooled in 1:1 mass ratios. All RNA extractions were done using Nucleospin RNA II (Macherey Nagel). RNA sequencing libraries were constructed to be sequenced on Illumina Hiseq 2000. See Supplementary Methods for details on library construction and Supplementary Table 12 for sequencing statistics. Genome assembly and annotation The velvet spider genome was assembled de novo using SOAPdenovo1 ( http://soap.genomics.org.cn ), which is based on transversing and pruning a de Bruijn graph. Low-quality reads were filtered out and potential sequencing errors were removed or corrected by the k-mer frequency methodology. The list of filters used can be found in Supplementary Methods . Assembly then proceeded with initial contig construction, followed by scaffolding and gap filling of the scaffolds. The tarantula genome was assembled de novo using SOAPdenovo 2 ( http://soap.genomics.org.cn ). Low-quality reads were filtered out before assembly using the same filtering criteria as for the velvet spider. Scaffolds were not gap-filled owing to the highly fragmented assembly. Genome assembly statistics are summarized in Supplementary Tables 13 and 14 . Gene models were constructed based on transcription evidence and on ab initio predictions. Approximately ~76 million paired-end reads were mapped to the 68,655 scaffolds from the velvet spider genome assembly using Tophat [56] . The alignments were analysed using Cufflinks [57] , producing 80,517 gene models. De novo -assembled transcripts were mapped to the genome using GMAP [58] to generate a second set comprising 28,684 models. The third set of gene models was produced using the ab initio gene predictor Augustus [59] , trained using the Cufflinks models, which resulted in 78,966 predicted protein-coding loci. The program parameters are summarized in Supplementary Table 15 . We refer to these three sets of gene models as Cufflinks, Velvet and Augustus, respectively. All three sets of gene models were then used separately as databases for protein identification based on the collected MS spectra. This allowed us to use a hierarchical selection scheme, taking proteomic support into account, to combine gene models from the three sources ( Supplementary Fig. 2 ) to a final set of 82,880 genes per loci and 87,438 gene models. Gene models were initially categorized according to Supplementary Fig. 12 , resulting in the distribution of protein-coding, repeat and unclassified models shown in Supplementary Table 2 . We then reviewed the degree of proteomics support for the different gene model categories. On average, the models classified as protein coding showed the highest level of support. However, the multi-exon unclassified gene models displayed a higher level of proteomics support than the single-exon gene models classified as protein coding. We therefore moved the unclassified multi-exon gene models and the unclassified single-exon models with proteomics support to the protein-coding gene category, resulting in a final gene set comprising 27,235 protein-coding genes and 31,745 gene models ( Supplementary Table 1 ). InterProScan [7] and BLAST against the UniRef100 database was used for gene annotation. See Supplementary Table 15 for parameter settings. Transcriptome assembly and annotation To reduce the amount of erroneous data, the raw paired reads from complementary DNA libraries were processed by (i) removing reads that contained the sequencing adaptor, (ii) removing reads that contained ambiguous characters (Ns) and (iii) trimming bases that had the low average quality (Q<20) within a sliding window of length 10. De novo assembly was performed using velvet (version 1.2.03) and Oases (version 0.2.06) with parameters 75-mer and ‘-ins_length 200 -ins_length_sd 10’. The assembly statistics results are shown in Supplementary Table 16 . The transcriptomes from the tarantula venom glands, opistosomal gland and soft tissue (except exoskeleton) were merged and translated. The longest open-reading frame sequences were identified and reported. To determine the function of protein sequences, we screened protein sequences against the non-redundant NCBI peptide database using Blastp with a cutoff e -value of 0.01. To assign proper annotation for each transcript, we chose the first best hit that was not represented in uninformative descriptions ( Supplementary Table 17 ). To specifically look for toxin sequences among the non-annotated sequences, these sequences were screened against the Arachnoserver-mygalomorphae toxin sequences using Blastp, which fulfilled the criteria that they were smaller than 10,000 dalton and contained >5 cysteines. Finally, the redundant protein sequences (identified using the CD-HIT Suite ( http://weizhong-lab.ucsd.edu/cdhit_suite/cgi-bin/index.cgi )) were removed. The final tarantula DNA sequences and the corresponding protein sequences can be found in Supplementary Data 3a, 3b and 4 . The predicted genes from the velvet spider were translated and the longest open-reading frame sequences were reported. Using the same strategy as for the tarantula, we assigned annotations of the protein sequences based on the NCBI non-redundant database. To specifically look for toxin sequences among the non-annotated sequences, these sequences were blasted against the Arachnoserver-araneomorphae toxin sequences, which fulfilled the criteria that they were smaller than 10,000 Da and containing >5 cysteines. The final velvet spider DNA sequences and the corresponding protein sequences can be found in Supplementary Data 5 and 6 . Genome characterization The exon-intron structure was determined by aligning all gene models to the assembly for the velvet spider. For the tarantula, the same overall idea was used but with mapping of the transcriptome assembly to the part of the genome included in scaffolds >100 kb, for a total of 0.65 Gb data. For the tarantula, repeat masking was done using RepeatModeler to build a de novo library of genomic repeats, and generated a library of 2,116 repeat sequences. Owing to the highly fragmented assembly, RepeatModeler was run on a subset of the assembly (120,425 scaffolds larger than 5,000 bp, covering a total of 4,142,570,934 bp). RepeatMasker was then used to repeatmask the entire assembly using this custom library and ignoring N/X runs. The genome of the velvet spider was analysed using a more detailed approach, made possible by the more complete assembly. First, we searched the genome for tandem repeats using Tandem Repeats Finder [60] . For interspersed repeats, we first used RepeatModeler to build a de novo repeat library, and generated a collection of 1,998 repeat sequences. Using this de novo repeat library as an input library, we ran RepeatMasker across the assembly. Besides repeat masking using a custom library, a combination of Repbase, plant repeat database and our genome de novo transposable element library, identified an additional 86 Mb repeat sequences. See Supplementary Methods for more details. GC content was calculated in 10-kb non-overlapping windows along both genomes ( Supplementary Fig. 13 ). Heterozygosities were found by aligning short reads against the assembled genome using bowtie2 (ref. 61 ) with the default parameters. The aligned reads were analysed by the widely used Genome-Analysis Toolkit (GATK, v2.0-39) [62] with default parameters to detect heterozygous SNPs. To guarantee the SNPs quality, we did local realignment and recalibrated the base quality as suggested by the manual of GATK. The above procedure identified 1,097,916 and 2,212,570 heterozygous SNPs in velvet spider and tarantula genomes, respectively. Overall, per nucleotide heterozygosity for velvet spider and tarantula are 0.021% and 0.34%, respectively. We also computed the folded site frequency spectrum based on the frequency of the minor allele at each locus for both velvet spider and tarantula SNPs ( Supplementary Fig. 14 ). Comparative genomics analysis Orthology between the velvet spider and the tarantula genes was determined by tblastx analysis with the similarity cutoff of e =1 e −5. Reciprocal best-match pairs were defined as orthologues. Non-synonymous (dN) substitution rates between all pairs of orthologues were estimated using the maximum-likelihood method implemented by CODEML [63] . See Supplementary Fig. 3 . Using the same method, we found 452 single-copy orthologues among velvet spider, tarantula, fruit fly, human, oyster, silkworm, spider mite and tick. We performed PRANK’s codon-based alignments [64] for each orthologue gene. Poorly aligned positions and divergent regions were removed using Gblocks in codon model [65] , [66] . Then, all well-aligned orthologue genes were concatenated to one super gene for one species. We translated the remaining high-quality coding sequences into amino-acid sequences and used PhyML [20] to construct the phylogenetic tree with the LG amino-acid substitution model. We also estimated the divergence time with approximate likelihood calculation implemented by PAML 4.7 MCMCtree using a relaxed-clock model with the following fossil times (MYA) as constraints [20] : velvet spider-tarantula: 235–396 (fossil Rosamygale), tick-spiders: 311–503 (oldest spider from coal, UK), spider mite+tick+spiders: 395–503 (oldest Acari), arthropods: 521–581, silkworm-fly: 239–295 (oldest dipteran), oyster-arthropods: 532–581 (oldest mollusk Latouchella) and human-all others (deuterostomes-protostomes: 519–581 (earliest vertebrate). We investigated gene family evolution by using Treefam’s [24] methodology to define a gene family as a group of genes that descended from a single gene in the last common ancestor of considered species, being the velvet spider ( Stegodyphus mimosarum ), the tarantula ( Acanthoscurria geniculata ), the tick ( Ixodes scapularis ), the spider mite ( Tetranychus urticae ), the fly ( Drosophila melanogaster ), the silkworm ( Bombyx mori ), the pacific oyster ( Crassostrea gigas ) and the human ( Homo sapiens ). Gene family expansion analysis was performed by CAFE 2.1 with all gene families. See Supplementary Methods for more details. SDS-PAGE and in-gel trypsin treatment Haemolymph, tissue samples, venom and silk samples were obtained as described in Supplementary Methods . A total of 6 mg lyophilized tarantula haemolymph, lyophilized tarantula tissues and homogenized velvet spider tissue were boiled in reducing, SDS-sample buffer, and subjected to SDS-PAGE using 5–15% (w/v) gradient gels and stained using Coomassie brilliant blue ( Supplementary Fig. 15 ). Similarly, the venom samples were subjected to SDS-PAGE. From the tarantula, the loaded amount per lane corresponded to 0.6 μl of crude venom, and from the velvet spider the total amount of venom from one individual was loaded (~0.2 μl) per gel lane ( Supplementary Figs 4 and 5 ). The gel lanes were sliced into pieces (in total 162 gel pieces, see Supplementary Table 3 ) and in-gel digestion with trypsin was essentially done as described before [67] . The resulting peptides were desalted using C 18 StageTips (Thermo Scientific) and stored at −20 °C before LC–MS/MS analysis. In-solution trypsin digestion of silk and venom Approximately 1 mg of silk was incubated with 1 ml 0.66 M cyanogen bromide in 70% trifluoroacetic acid overnight at 23 °C. Subsequently the sample was lyophilized and the remaining pellet dissolved in 1 ml 100% formic acid and incubated for 23 °C for 1 h. Then the sample was lyophilized and dissolved in ammonium bicarbonate and lyophilized again. Afterwards, the proteins were dissolved in a reducing, 8M urea buffer and subsequently alkylated using iodoacetamide. The sample was then diluted with ammonium bicarbonate buffer and digested with trypsin (Promega) for 16 h at 37 °C. The sample was desalted using R2-material (PerSeptive Biosystems) packed in gel-loading tips, and stored at −20 °C before LC–MS/MS analysis. The described protocol was applied to all silk samples. After the described treatment, a pellet remained in the test tubes, suggesting that the procedure did not completely dissolve the silk. Thus, we also tested an alternative protocol, which included extensive sonication and treatment of the silk with 100% hexafluoroisopropanol at 37 °C, rotating, overnight as an initial step, in addition to the steps described above. However, a pellet was also present after this procedure, and consequently hexafluoroisopropanol was omitted, and the procedure described above was used. With regard to venom, it was not possible to obtain sufficient material for LC-MS/MS analyses on individual velvet spiders. Therefore, venom from three individual spiders was pooled for the in-solution trypsin digestion of venom proteins. The two spider species were treated identical and the venom from the three tarantulas was similarly pooled. The in-solution trypsin digestion of the venom proteins were performed after reduction and alcylation in 8 M urea, as described for the silk samples. The resulting peptides were desalted using C 18 StageTips (Thermo Scientific) and stored at −20 °C before LC–MS/MS analysis. LC–MS/MS analyses and protein identification LC–MS/MS analyses were performed on an EASY-nLC II system (Thermo Scientific) connected to a TripleTOF 5600 mass spectrometer (AB Sciex) equipped with a NanoSpray III source (AB Sciex) and operated under Analyst TF 1.6 control. See Supplementary Methods for further details. In total, 194 LC-MS/MS analyses were performed ( Supplementary Table 3 ). The MS proteomics data have been deposited to the ProteomeXchange Consortium ( http://proteomecentral.proteomexchange.org ) via the PRIDE partner repository with the data set identifier PXD000318 and DOI 10.6019/PXD000318 (ref. 68 ). The generated peak lists were used to interrogate the produced spider-protein databases using Mascot 2.3.02 (Matrix Science) [69] . The criteria for protein identification are detailed in Supplementary Methods . The Mascot results were subsequently parsed using MS Data Miner v. 1.1.3 (ref. 70 ), and protein hits were only accepted if they were identified based on two unique peptides. The only exceptions from this criterion were the identification of (i) the cysteine-rich peptide toxins, (ii) proteins for gene-prediction support and (iii) the velvet spider spidroins. These exceptions are described in detail in Supplementary Methods and Supplementary Table 6 . The full list of identified proteins and the peptides used for identification can be found in Supplementary Data 1 and 2 . Extracted-ion chromatography-based protein quantification The LC-MS/MS analyses of in-solution digests of venom and silk (except dragline and egg case silk) were used for XIC quantification (see Supplementary Methods for details on the samples, settings and criteria). Mascot Distiller 2.4.3.3 (Matrix Science) was employed for these analyses and the resulting xml files were imported and processed using MS Data Miner [70] . The relative abundance of proteins quantified was calculated as the average MS intensity for the three most intense peptides for each protein divided by the total sum of the average signal for all quantified proteins in the sample. As described in Supplementary Methods , a pellet is left after trypsin treatment of silk and therefore the silk protein quantification should be taken with precaution. The relative small size of the peptide toxins in venom, results in a limited number of potential tryptic peptides suited for the MS instrument. Consequently, the quantification of these toxins, based on three quantifiable tryptic peptides, is difficult for many of these sequences. Therefore, the quantification of venom components is, in the present study, split in two different analyses: one focusing on the protein content of venom, and one focusing on the cysteine-rich peptide toxins. The XIC approach was used for quantification of the venom proteins and spectral counting was used for quantification of the protoxins. The protoxins that were present on the XIC-derived list of venom components were manually removed, and the relative protein abundance was re-calculated after manual removal of the toxin sequences. Spectral counting-based protein quantification The quantification of Dragline silk (velvet spider), Egg case silk (velvet spider) and toxins (both spiders) were based on spectral counting. The analyses of Dragline and Egg case silk were based on a single LC-MS/MS analysis, whereas the toxin analyses are based on four technical replicas for the tarantula and eight technical replicas for the velvet spider. The technical replicas were merged into a single file (for each species), which were used to query the toxin databases (see Supplementary Note 2 ). The resulting files were sorted according to the significant matches, which represents the total number of times that MS/MS spectra have been generated for peptides belonging to a given protein. The quantitative proteomics data, both based on XIC and spectral counting, are included in Supplementary Data 7 and 8 . Accession Codes . Raw sequencing data have been deposited in the Genbank/EMBL/DDBJ sequence read archive (SRA) under the accession codes SRA106216 (tarantula) and SRA106215 (velvet spider). Spider genome assemblies have been deposited in the Genbank/EMBL/DDBJ BioProjects database under the accession codes PRJNA222716 (tarantula) and PRJNA222714 (velvet spider). Assembled transcriptomes have been deposited in the Genbank/EMBL/DDBJ Transcriptome Shotgun Assemblies (TSA) database under the accession codes GAZS00000000 (tarantula) and GAZR00000000 (velvet spider). How to cite this article: Sanggaard, K. W. et al. Spider genomes provide insight into composition and evolution of venom and silk. Nat. Commun. 5:3765 doi: 10.1038/ncomms4765 (2014).